Aedes aegyptiArgonaute 2 controls arbovirus infection and host mortality Ae. aegypti mosquitoes transmit some of the most important human viral diseases that are responsible for a significant public health burden worldwide. The small interfering RNA (siRNA) pathway is considered the major antiviral defense system in insects. Here we show that siRNA pathway disruption by CRISPR/Cas9-based Ago2 knockout impaired the mosquitoes’ ability to degrade arbovirus RNA leading to hyper-infection accompanied by cell lysis and tissue damage. Ago2 disruption impaired DNA repair mechanisms and the autophagy pathway by altering histone abundance. This compromised DNA repair and removal of damaged cellular organelles and dysfunctional aggregates promoted mosquito death. We also report that hyper-infection of Ago2 knockout mosquitoes stimulated a broad-spectrum antiviral immunity, including apoptosis, which may counteract infection. Taken together, our studies reveal novel roles for Ago2 in protecting mosquitoes from arbovirus infection and associated death. The yellow fever mosquito Aedes aegypti is the principal vector of numerous medically important human pathogens, including dengue virus (DENV), Zika virus (ZIKV), chikungunya virus (CHIKV) and Mayaro virus (MAYV). These pathogens are transmitted between humans and mosquitoes and represent a major public health causing socioeconomical burden globally [1] , [2] . The populations at risk of mosquito-borne diseases have grown substantially in recent years and could potentially extend to low-risk countries in Asia, Europe and North America because of the spread of Aedes mosquito vectors as a result of climate change [3] , [4] , [5] . Current methods to control mosquito-borne diseases that have emerged, or re-emerged, in many geographical regions are proving insufficient because of insecticide resistance and a lack of effective vaccines. Vector control remains the principal method for controlling and limiting mosquito-borne diseases [6] . In recent years, with the development of genome editing and mosquito transgenesis, novel control strategies based on population suppression or population replacement have been proposed as alternatives for the control of mosquito-borne diseases [7] . To defend against infection with arboviruses, mosquitoes use their innate immune system, which includes the small interfering RNA (siRNA) pathway, Toll pathway, JAK/STAT pathway, and other defenses [8] , [9] . These innate immunity pathways control systemic infection in mosquitoes by maintaining arbovirus infection intensity at a level that does not cause pathogenesis in the mosquitoes but still enables the transmission of the pathogens [10] . This balance is crucial for vector competence for arboviruses. Otherwise, mosquitoes would suffer a high fitness cost because of virus infection and likely evolve total refractoriness to infection, which would not enable the viruses to be transmitted. The siRNA pathway is the major antiviral defense system against arbovirus infections in Ae. aegypti and plays an important role in maintaining the mosquito-arbovirus balance [11] , [12] . The core components of the siRNA pathway include the RNase III enzyme Dicer 2 (Dcr2), a dsRNA-binding protein (dsRBP) called R2D2, and the endoribonuclease Argonaute 2 (Ago2) [13] , [14] , [15] . Double-stranded viral RNA is first recognized and digested by Dcr2 into 21 nt-siRNAs. These viral siRNAs are then incorporated into the RNA-induced silencing complex (RISC) with the integration of R2D2, leading to the degradation of the viral RNAs by Ago2. Ago2 is a member of the evolutionarily conserved Argonaute family, whose members feature typical PIWI and PAZ domains. In addition to the essential role of Ago2 in regulating gene silencing in the cytoplasm, this enzyme has been shown to regulate gene expression in the nucleus [16] , [17] and to play a role in translation repression and heterochromatinization [18] . Ago2 interacts with LaminB, a nuclear scaffolding protein, to form a nuclear complex and modulate chromatin topology in Drosophila melanogaster [19] . To date, functions of Ago2 beyond its involvement in the siRNA pathway have not been explored in any mosquito species. In Drosophila , a defective siRNA pathway impairs the flies’ ability to defend against viral infection, resulting in high mortality [14] , [15] . However, most data derived from experiments using Drosophila -virus models are based on artificial infections in which the virus is injected into the insect [14] , [20] . This injection approach does not reflect the natural infection cycle of arboviruses that are initiated through virus acquisition through an infected blood meal, after which the viruses infect the midgut tissue before being disseminated to other tissues [21] . Furthermore, the viruses used for Drosophila infection studies are different from those causing mosquito-borne human diseases such as dengue, Zika, yellow fever, Mayaro, and chikungunya [22] . Therefore, to study the role of the siRNA pathway in controlling arbovirus infection in mosquitoes, we have now generated siRNA pathway-defective mosquitoes by knocking out Ago2 in Ae. aegypti . Our study shows a fundamental role for Ago2 and the siRNA pathway in controlling arbovirus infection in mosquitoes, as well as in protecting the mosquitoes against mortality upon arboviral infection by modulating DNA repair, apoptosis, and autophagy. Our study provides insights into the molecular interactions between mosquitoes and arboviruses that may facilitate the development of novel disease control strategies. Generation and characterization of Ago2 knockout mutants To demonstrate the essential function of Ago2 in the Ae. aegypti siRNA pathway, we used CRISPR/Cas9 to knock out Ago2 and then investigated its role in defending against arbovirus infection (Fig. 1a ). Ae. aegypti Ago2 ( AeAgo2 ) has four exons and four predicated functional domains, and its PAZ and Piwi_Ago-like domains are considered essential for endonuclease activity (Fig. 1b and Supplementary Fig. 1a ). Therefore, we designed guide RNAs (gRNAs) targeting the Piwi_Ago-like domain encoded by exon 3. Meanwhile, another two gRNAs targeting the ArgoN domain encoded by exon 1 were designed and used to induce frameshift mutations that resulted in Ago2 disruption. Through embryo injection and leg PCR screening, we generated at least two independent Ago2 knockout mutant lines: one line ( ArgoN −/− ) with a mutation in exon 1 and another line ( Ago2 −/− ) with a mutation in exon 3 (Fig. 1c and Supplementary Fig. 1b ). ArgoN −/− has a frameshift mutation (a 51-bp deletion and 14-bp insertion) in the first reading frame but uses the second reading frame to translate a truncated protein (Supplementary Fig. 1c ). Ago2 −/− line has an in-frame mutation with a 72-bp deletion in the Piwi_Ago-like domain. Fig. 1: Generation of Ago2 knockout Ae. aegypti lines and the effect of Ago2 disruption on arbovirus infection and transmission. a flowchart of experiment design. b gene structure of Ago2 , predicted functional domains, and guide RNA (gRNA) design for CRISPR/Cas9. The table shows data from generating Ago2 knockout lines. c Ago2 amplification in Ago2 knockout lines. P, parental line Cas9 ; HE, heterozygous mutants; HO, homozygous mutants. d virus titer in Ago2 knockout ( Ago2 −/− and ArgoN −/− ) and Cas9 mosquitoes on various days post-infection (dpi) with DENV2, ZIKV, or MAYV. IFA detection of MAYV ( e ) and DENV2 ( f ) antigen in midguts of Cas9 and Ago2 −/− mosquitoes at different days post virus infection. MAYV and DENV2 were detected with the corresponding monoclonal antibody (green). Nuclei were stained with DAPI (blue). g virus titer and infection prevalence in the feeding solution collected from a feeder exposed to a group of females at 14 dpi with DENV2 or 5 dpi with MAYV. The Liverpool strain was used as a control (WT). For DENV2 infection, n = 16 for WT and n = 15 for Ago2 −/− ; for MAYV infection, n = 19 for both WT and Ago2 −/− . h percentage of the fed mosquitoes in each group of females at 14 dpi with DENV2 or 5 dpi with MAYV. Data were presented as box and whiskers (Min to Max). i virus titer plotted against the number of the fed mosquitoes in each cup. j virus titer and infection prevalence of individual saliva samples collected from Ago2 −/− and WT at 14 dpi with DENV2 or 5 dpi with MAYV. For DENV2 infection, n = 62 for WT and n = 61 for Ago2 −/− ; for MAYV infection, n = 56 for both WT and Ago2 −/− . Each experiment comprised at least two biological replicates, and the data were pooled for generating the graphs. Virus titers were determined by plaque assay, and horizontal lines indicate the medians of the virus titer ( d , g and j ). P values were determined by an unpaired two-sided Mann-Whitney test for virus titer, an unpaired two-sided Fisher’s exact test for infection prevalence, or an unpaired two-sided t -test for ( h ). Source data are provided as a Source Data file. Full size image To assess whether the siRNA pathway was impaired in Ago2 knockout mutant lines, we performed three independent assays of RNA interference-based silencing different endogenous genes in WT and Ago2 knockout mutants. (1) We attempted silencing of the kynurenine hydroxylase ( kh ) gene (AAEL008879) in embryos of WT and Ago2 −/− and AgoN −/− mutants through microinjection of kh dsRNA. The kh gene is essential for the kynurenine 3-monoxygenase (KMO) function which is critical for eye pigmentation, and knockout of the kh gene leads to severe eye pigmentation defects [23] . As compared to the GFP dsRNA-injected control, a serious defect in eye pigmentation was observed in 3rd instar larvae hatched from kh dsRNA-injected WT eggs, however, we did not observe any defect in eye pigmentation in larvae hatched from kh dsRNA-injected Ago2 −/− eggs (Supplementary Fig. 1d ). We observed a mild defect in eye pigmentation in larvae hatched from kh dsRNA-injected AgoN -/- eggs. These results indicated that the Ago2 -/- mutant is completely defective of the siRNA function, therefore a Ago2 null mutant, while the AgoN −/− mutant still has some residual siRNA function, therefore a partially Ago2 knockout mutant. (2) We attempted silencing of the eggshell organizing factor 1 ( EOF1 ) gene (AAEL012336) in WT and Ago2 −/− females through injection of EOF1 dsRNA . EOF1 plays an essential role in the formation and melanization of the eggshell and silencing of EOF1 leads to a defect in eggshell melanization and reduction in fecundity [24] . EOF1 dsRNA-injected WT females produced significantly less eggs and eggs showed defects in eggshell melanization when compared to the GFP dsRNA-injected control, however, EOF1 dsRNA-injected Ago2 −/− females did not show any difference in fecundity and eggshell melanizaiton as compared to the GFP dsRNA-injected controls (Supplementary Fig. 1e ). (3) We attempted silencing of three genes ( AeIMPDH , AeCRVP and AeTry196 ) that had been reported to show significant silencing through dsRNA injection in our previous studies [25] , [26] . Compared to WT where gene silencing was significant, Ago2 −/− mutants didn’t show gene silencing (Supplementary Fig. 1f ). Taken together, our data demonstrate that RNAi-mediated silencing is fully abolished in the Ago2 −/− mutants. Multiple fitness parameters were assayed in WT and Ago2 −/− mutants. The results showed that there were no differences in whole-body weight (Supplementary Fig. 2a ), amount of ingested blood (Supplementary Fig. 2b ), percentage of blood-fed mosquitoes (Supplementary Fig. 2c ) and fertility of eggs between the WT and Ago2 −/− mutants (Supplementary Fig. 2f ). However, the Ago2 −/ − mutants have a significantly delayed larva development (Supplementary Fig. 2d ), a reduced fecundity (Supplementary Fig. 2e ) and a shorter life span of females and males (Supplementary Fig. 2g ). Ago2 is required for controlling arboviral infection in mosquitoes, and Ago2 disruption reduces arbovirus transmission We performed independent natural infections of various Ago2 knockout mutant lines and the control (the parental Cas9 line) mosquitoes with different arboviruses, including two flaviviruses (DENV2 and ZIKV) and one alphavirus (MAYV) through blood meal. As compared to the control Cas9 mosquitoes, both ArgoN −/− and Ago2 −/− mutants exhibited a significantly higher titer of each of the three tested viruses, when measured at 14 days post-infection (dpi) for DENV2 and ZIKV and at 7 dpi for MAYV (Fig. 1d ). At earlier time points, the virus titer was not significantly different between ArgoN −/− mutants and the control mosquitoes : at 7 dpi in the case of DENV2 and 3 dpi in the case of MAYV, however, the virus titer in Ago2 −/− mutants was significantly higher than that of the Cas9 controls at both the early and late time points for all three viruses. Hence, a mutation in the Piwi_ago-like domain had the strongest impact on arbovirus infection and Ago2 endonuclease activity, which was also shown in dsRNA-mediated silencing of endogenous genes (Supplementary Fig. 1d ), and the Ago2 −/− line was therefore used as a Ago2 mutant line for the subsequent experiments. Midguts of Ago2 −/− females displayed a different infection pattern upon arbovirus infection: for MAYV at 4 dpi, the infection of the control midgut was restricted to specific areas, whereas half the Ago2 −/− midgut was heavily infected (Fig. 1e ). At 7 dpi, the whole midgut of Ago2 −/− females was strongly infected by MAYV, and the midguts also assumed a rounder shape than those of the Cas9 midguts. At 7 dpi and 14 dpi with DENV2, a more intense infection was observed in midguts of Ago2 −/− females when compared to those of the Cas9 midguts (Fig. 1f ). The tracheas associated with midguts were heavily infected by MAYV or DENV2 in Ago2 −/− mutants when compared to the control mosquitoes (Supplementary Fig. 3 ). These data demonstrate that Ago2 plays an essential role in controlling virus infection intensity in Ae. aegypti and mosquitoes become hypersensitive to arbovirus infection when Ago2 is disrupted. To determine the effect of Ago2 disruption on the transmission potential of arboviruses, we examined the levels of virus particles released into the feeding solution from the proboscises of arboviruses-infected Ago2 −/− and WT females through an artificial feeding system. As compared to the WT females, Ago2 −/− females exhibited a significant reduction of virus particles released into the feeding solution at 14 dpi with DENV2 or 5 dpi with MAYV, and only 4 of 15 feeding solution samples collected from the feeders were positive for DENV2 and 3 of 19 were positive for MAYV after exposure to Ago2 −/− females, but 14 of 16 feeding solution samples were positive for DENV2 (Fig. 1g ). In contrast, all feeding solution samples exposed to infected WT females were positive for MAYV (Fig. 1g ). We also investigated whether arbovirus-infected Ago2 −/− females displayed any altered feeding propensity (the portion of the fed mosquitoes), and we found that the number of either DENV2- or MAYV-infected Ago2 −/− females that had fed was significantly lower than that of the WT mosquitoes (Fig. 1h ). We could not detect any DENV2 or MAYV in the feeding solution of some groups of virus-infected Ago2 −/− mosquitoes that were fed (Fig. 1i ), suggesting that some Ago2 −/− mutants may fail to release virus into their saliva. To further examine this, we used a forced-salivation method to compare the number of viral particles released in the saliva of Ago2 −/− and WT females at 14 dpi with DENV2 or 5 dpi with MAYV. We found no significant difference in the virus titer in the saliva samples from Ago2 −/− mutants and WT mosquitoes for both DENV2 and MAYV, but the Ago2 −/− mutants showed a significantly reduced virus prevalence (i.e., a reduced proportion of mosquitoes having virus particles in the saliva; Fig. 1j ). Taken together, these data indicate that Ago2 disruption significantly reduces the arbovirus transmission potential of mosquitoes by affecting the feeding propensity and the shedding of virus particles into the saliva from the salivary glands. Ago2 is not required for small RNA biogenesis in mosquitoes, but Ago2 disruption impairs viral RNA degradation To determine whether the effect of Ago2 disruption on arbovirus infection was the result of a defective siRNA pathway, we performed small RNA (sRNA) sequencing of Ago2 −/− mutants and WT mosquitoes after MAYV infection. At 4 dpi with MAYV, a significantly higher number of MAYV sRNA was observed in Ago2 −/− mutants as compared to the WT mosquitoes (Fig. 2a ). qPCR analyses showed that the MAYV titer in Ago2 −/− mutants was significantly higher than that in the WT mosquitoes (Supplementary Fig. 4a ), and a principal component analysis (PCA) indicated that the high yield of vsRNAs could be explained by the high virus titer in Ago2 −/− mutants (Fig. 2b ). The length of the viral sRNAs (vsRNAs) was distributed between 18 nt and 40 nt with a dominant peak at 21 nt at 4 dpi with MAYV in both Ago2 −/− mutants and WT mosquitoes (Fig. 2c ), demonstrating that Ago2 −/− mutants still produced 21 nt-biased vsRNAs. Ago2 −/− mutants also produced a number of non 21-nt vsRNAs (Fig. 2c ), and these vsRNAs had a prominent positive-strand bias (Supplementary Fig. 4b ). Fig. 2: Impact of Ago2 disruption on production of MAYV- and mosquito-derived small RNAs. a total number (reads per million mapped reads, RPM) of MAYV sRNAs in Ago2 −/− mutants and WT mosquitoes at 4 days post-infection (dpi) as determined by sRNA sequencing. Three replicates were performed for each sample. b correlation between the abundance of sRNAs and titer of MAYV in Ago2 −/− mutants and WT mosquitoes as determined by principal component analysis (PCA). c distribution by length of sRNAs mapping to the MAYV genome. d number of 21-nt siRNAs mapped to the MAYV genome. e the ratio of siRNA-sized (21 nt) MAYV reads to the total MAYV sRNA (18nt to 40nt) reads. f distribution and the relative abundances of 21-nt MAYV siRNAs in the MAYV genome. g number of total sRNAs mapped to the Ae. aegypti genome. h percent of MAYV sRNAs in the total sRNAs in mosquitoes. i number of 21-nt siRNAs mapped to the Ae. aegypti genome. j length distribution of the mosquito sRNAs. P values were determined by using an unpaired two-sided t -test ( n = 3) with GraphPad Prism. Data are presented as mean ± SEM ( a , d and e ). Source data are provided as a Source Data file. Full size image Since the biogenesis of vsRNA was not affected by Ago2 disruption, we investigated whether the number of 21 nt viral small interfering RNAs (vsiRNAs) that bound to siRNA pathway factors was altered in Ago2 −/− mutants. A higher number of MAYV vsiRNA was observed in Ago2 −/− mutants as compared to WT mosquitoes (Fig. 2d ), but the ratio of vsiRNA reads to the total vsRNA reads was lower in Ago2 −/− mutants (Fig. 2e ) because they produced a greater number of non-21nt-vsRNA as compared to WT mosquitoes (Fig. 2b ). There was a similar distribution of 21 nt vsiRNA in the positive or negative strand of the MAYV genome between Ago2 −/− mutants and WT mosquitoes, but the relative abundances of the vsiRNAs were different because of the higher vsRNA reads in Ago2 −/− mutants (Fig. 2f ). Therefore, our results show that Ago2 disruption does not affect the production of arboviral sRNAs but does impair the ability of the siRNA pathway to degrade viral RNAs, as reflected by a high virus titer and an impaired RNA silencing in Ago2 −/− mutants. The total sRNAs were also mapped to the Ae. aegypti genome. The results showed that Ago2 disruption significantly reduced the abundance of the mosquito sRNAs at 4 dpi with MAYV (Fig. 2g ), likely because of a higher fraction of MAYV sRNAs in the total sRNAs in Ago2 −/− mutants (Fig. 2h ). As compared to WT mosquitoes, Ago2 −/− mutants produced a higher number of mosquito 21 nt siRNAs (Fig. 2i ), suggesting that Ago2 disruption may increase the abundance of the mosquito endogenous dsRNAs. The length distribution of the mosquito sRNAs showed no difference between Ago2 −/− mutants and WT mosquitoes, and both showed two peaks at 21–23 and 26–30 nt, corresponding to microRNAs and piwiRNAs, respectively (Fig. 2j ). To further determine the influence of the Ago2 disruption on the mosquito’s ability to degrade arbovirus RNA, we performed independent sRNA sequencing on another Ago2 mutant line ( ArgoN −/− ) and its parental line ( Cas9 ) at 2 dpi and 7 dpi with DENV2. The sRNA sequencing results of DENV2-infected ArgoN −/− mutants were very similar to what we observed in MAYV-infected Ago2 −/− mutants, including a significantly higher number of total DENV2 sRNA (Supplementary Fig. 4c, d, e ), 21nt DENV2 siRNA (Supplementary Fig. 4f, g ), total mosquito sRNA (Supplementary Fig. 4h ), and 21 nt mosquito siRNA reads (Supplementary Fig. 4i ), and no difference in length distribution of the mosquito sRNAs (Supplementary Fig. 4j ) in ArgoN −/− mutants as compared to the Cas9 mosquitoes, and the high yield of DENV2 vsRNAs could be resulted from the high virus titer in ArgoN −/− mutants (Supplementary Fig. 4k ). Overall, our studies have shown that Ago2 disruption does not affect the biogenesis of sRNAs in either arboviruses or mosquitoes and the increased abundance of viral sRNAs that we found is due to the high arbovirus titer in Ago2- deficient mosquitoes. Arbovirus infection results in high mortality of Ago2 -deficient mosquitoes through cell lysis To determine whether hyper-infection of arboviruses can lead to the death of Ago2 −/− mutants, we performed a mortality assay involving DENV2, ZIKV, and MAYV infections transmitted through oral blood-feeding as well as through direct injection of viruses into the mosquito hemolymph. Our results showed that Ago2 −/− mutants experienced a significantly higher mortality upon infection with the three different arboviruses than did WT mosquitoes infected through the two different infection routes, but direct injection of the viruses resulted in higher mortality than did natural infection through blood-feeding (Fig. 3a ). Of all the arboviruses we tested, MAYV infection resulted in the highest mortality of Ago2 −/− mutants (Supplementary Fig. 5a ), and the median survival after MAYV infection was 6 days for the orally infected and 4 days for the virus-injected Ago2 −/− mutants (Fig. 3a ); therefore, Ago2 −/− mutants and MAYV infection were used for the future experiments to explore the mechanism of arbovirus-induced mortality of Ago2 −/− mutants. Arbovirus infection also caused the mortality of ArgoN −/− mutants, a mutation in the ArgoN domain of Ago2, but it is lower than that of Ago2 −/− mutants (Supplementary Fig. 5b ); these results were correlated with the virus titer in the various Ago2 knockout mutant lines (Fig. 1d ), suggesting that the high mortality of the Ago2 −/− mutants may be a result of their high infection intensity. The virus infection intensity-dependent mortality was then confirmed through injection of different titers of MAYV into Ago2 −/− mutants where a higher titer of MAYV led to higher mortality of Ago2 −/− mutants (Supplementary Fig. 5c ). Fig. 3: Effect of arbovirus infection on mosquito death and tissue/cell damage in Ago2 −/− mutants. a survival curves of Ago2 −/− and wild-type (WT) females that ingested a blood meal containing DENV2, ZIKV, or MAYV or were mock-infected (given C6/36 cell culture medium), or were injected with DENV2, ZIKV, or MAYV or mock-infected medium. P values between Ago2 −/− mutants and WT mosquitoes were determined using the logrank (Mantel-Cox) test. Each experiment comprised at least three biological replicates. The error bands were indicated by the shaded region. IFA detection with the anti-MAYV monoclonal antibody (green) of MAYV in midguts ( b ) and salivary glands ( c ) of Ago2 −/− and WT females at various days post-infection (dpi). Nuclei were stained with DAPI (blue). The zoomed areas are indicated as white boxes and arrows. White arrows indicate abnormal nuclei, and red arrows indicate strong fluorescence with a “ball” shape. Ultrastructural TEM images showing cross-sections of midgut tissue of Ago2 −/− mutants and WT mosquitoes at 4 dpi ( d ) and 7 dpi ( e ) with MAYV. Yellow arrows indicate individual virion; white dotted lines outline a cluster of virions. Scale bars are indicated on each image. Abbreviations: BL basal lamina, nc nucleus. The IFA and TEM images in ( b – e ) are representative of three biologically independent samples. Source data are provided as a Source Data file. Full size image We also used IFA to examine the infection of the midguts and salivary glands of Ago2 −/− mutants and WT mosquitoes after MAYV and DENV2 infection. At 4 dpi with MAYV, the midguts of the Ago2 −/− females showed a strong fluorescence with a “ball”-like shape that comprises hyper-infected midgut cells, indicating that the insects were hyper-infected by viruses (Fig. 3b ), and the nuclei of a large proportion of the midgut cells were highly condensed and exhibited an abnormal shape when compared to those of the WT midguts (Fig. 3b ); these findings suggested that the cells of Ago2 −/− mutants were likely undergoing lysis as a consequence of virus hyper-infection. At 7 dpi with MAYV, the infection and lysis of midgut epithelial cells were even higher in Ago2 −/− females, and most of the midgut cells were lysed (Fig. 3b ). At 7 dpi and 14 dpi with DENV2, the higher infection and lysis of the midgut epithelial cells were also observed in Ago2 −/− females when compared to the WT midguts (Supplementary Fig. 5d ). A similar pattern of condensed nuclei and hyper-infection was observed in the salivary glands of Ago2 −/− females upon MAYV infection (Fig. 3c ), suggesting that cell lysis might occur in multiple tissue and cell types in Ago2 −/− mutants in response to arbovirus infection. We did not observe lysis of midguts and salivary glands in uninfected Ago2 −/− mutants as compared to the WT mosquitoes (Supplementary Fig. 5e ). The virus -induced lysis of salivary gland cells is likely to have affected the shedding of viral particles into the saliva, leading to the observed reduction in feeding and arboviral transmission by the Ago2 −/− mutants (Fig. 1h, j ). We then employed transmission electron microscopy (TEM) to examine the cell lysis in the midguts of Ago2 −/− females upon arbovirus infection. Ultrastructural studies showed that the nuclei of the Ago2 −/− midgut cells displayed an elongated shape, and the nucleolus was not well formed at 4 dpi with MAYV, compared to the WT midgut cells (Fig. 3d ), indicating that the cells may undergo nuclear fragmentation and apoptosis. Moreover, clusters of virions were observed in the midgut cells of Ago2 −/− mutants, whereas the virions were evenly distributed in the WT midguts. At 7 dpi with MAYV, the pattern of infection in the WT midguts was similar to that at 4 dpi, but more virions were observed; in contrast, the midgut epithelial cells of Ago2 −/− females were completely lysed and devoid of nuclei, and the virus particles appeared to be present throughout the entire cell (Fig. 3e ). In summary, our data demonstrate that Ago2 −/− mutants have a weakened defense against arbovirus infection and that hyper-infection lyses the mutant mosquitoes’ cells and damages their tissues, leading to pathogenesis that compromises their feeding propensity (Fig. 1h ) and viability (Fig. 3a ). Arbovirus hyper-infection stimulates broad-spectrum antiviral immunity in Ago2 -deficient mosquitoes To probe to the underlying mechanism governing the infection-induced mortality in Ago2 −/− mutants, we compared the whole transcriptomes of MAYV-infected Ago2 −/− and WT females, as well as uninfected Ago2 −/− and WT females. As compared to the WT mosquitoes, we found that 1,279 genes were upregulated, and 1,128 genes were downregulated in Ago2 −/− mutants in response to MAYV infection at 4 dpi (Fig. 4a and Supplementary Data 1 ), and 555 upregulated and 280 downregulated genes in uninfected Ago2 −/− mutants (Supplementary Data 2 ). Fig. 4: Transcriptomic analysis of antiviral immune signaling in Ago2 −/− mutants upon MAYV infection. a flowchart illustrating the design and outcome of RNAseq experiments comparing transcriptome changes in Ago2 −/− mutants and WT mosquitoes. DE genes, differentially expressed genes. n = 3 biological replicates. b interaction network illustrating the upregulated gene families in Ago2 −/− mutants. The light color indicates the small P -value (one-sided Fisher’s exact test), and the small size of the bubble indicates the few genes in the GO term. The immunity- and defense-related GOs are indicated by asterisks. c fold enrichment of the significantly upregulated gene families in Ago2 −/− mutants. The immunity-related gene families are outlined red. d heatmap illustrating transcriptome changes in the upregulated immunity genes in Ago2 −/− mutants. e detection of caspase activity in midguts of Ago2 −/− and WT females. Data are presented as mean ± SD ( n = 4). f confirmation by qPCR of the upregulated expression of caspase and apoptosis genes in midguts of Ago2 −/− females. Data are presented as mean ± SD ( n = 4). g TUNEL assay to detect apoptotic cells (red) in midguts of Ago2 −/− and WT females. MAYV antigen is indicated by green, and nuclei are in blue. h survival curves for the MAYV-infected WT females that were fed with apoptosis inducer PAC-1 or apoptosis inhibitor Z-VAD-FMK (VAD) or an equal amount of DMSO in 10% sucrose solution. Data are presented as percents ± SE ( n = 3). i virus titer in WT females treated with PAC-1 or VAD at 7 dpi with MAYV. Data were presented as box and whiskers (Min to Max), n = 30. j upregulated immune genes related to B-cell, T-cell, complement (Suchi), or macroglobulin (Mg) in Ago2 −/− mutants. k upregulated immunoglobulin (Ig)-like genes in Ago2 −/− mutants. P values were determined by one-way ANOVA ( e and f ), an unpaired two-sided Mann-Whitney test ( i ), or a logrank (Mantel-Cox) test ( h ). Source data are provided as a Source Data file. Full size image GO and interacting network analysis of the upregulated genes showed an enrichment of mRNAs corresponding to genes with predicted functions in the categories of immune response, defense, and response to stimuli in Ago2 −/− mutants at 4 dpi with MAYV when compared to the WT mosquitoes (Fig. 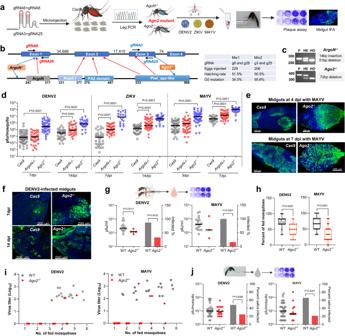Fig. 1: Generation ofAgo2knockoutAe. aegyptilines and the effect ofAgo2disruption on arbovirus infection and transmission. aflowchart of experiment design.bgene structure ofAgo2, predicted functional domains, and guide RNA (gRNA) design for CRISPR/Cas9. The table shows data from generatingAgo2knockout lines.cAgo2amplification inAgo2knockout lines. P, parental lineCas9; HE, heterozygous mutants; HO, homozygous mutants.dvirus titer inAgo2knockout (Ago2−/−andArgoN−/−) andCas9mosquitoes on various days post-infection (dpi) with DENV2, ZIKV, or MAYV. IFA detection of MAYV (e) and DENV2 (f) antigen in midguts ofCas9andAgo2−/−mosquitoes at different days post virus infection. MAYV and DENV2 were detected with the corresponding monoclonal antibody (green). Nuclei were stained with DAPI (blue).gvirus titer and infection prevalence in the feeding solution collected from a feeder exposed to a group of females at 14 dpi with DENV2 or 5 dpi with MAYV. The Liverpool strain was used as a control (WT). For DENV2 infection,n= 16 for WT andn= 15 forAgo2−/−; for MAYV infection,n= 19 for both WT andAgo2−/−.hpercentage of the fed mosquitoes in each group of females at 14 dpi with DENV2 or 5 dpi with MAYV. Data were presented as box and whiskers (Min to Max).ivirus titer plotted against the number of the fed mosquitoes in each cup.jvirus titer and infection prevalence of individual saliva samples collected fromAgo2−/−and WT at 14 dpi with DENV2 or 5 dpi with MAYV. For DENV2 infection,n= 62 for WT andn= 61 forAgo2−/−; for MAYV infection,n= 56 for both WT andAgo2−/−. Each experiment comprised at least two biological replicates, and the data were pooled for generating the graphs. Virus titers were determined by plaque assay, and horizontal lines indicate the medians of the virus titer (d,gandj).Pvalues were determined by an unpaired two-sided Mann-Whitney test for virus titer, an unpaired two-sided Fisher’s exact test for infection prevalence, or an unpaired two-sidedt-test for (h). Source data are provided as a Source Data file. 4b and Supplementary Table 1 ). A group of immune genes, including caspases, C-type lectin (CTL), and leucine-rich repeat (LRR) family members was significantly enriched in Ago2 −/− mutants (Fig. 4c and Supplementary Data 1 ). Most of the upregulated immune genes such as genes from the CTL, fibrinogen-related protein (FREP), Clip-domain serine protease (CLIP) and peptidoglycan recognition protein (PGRP) family have immune-defense/antibacterial functions, but two groups of genes (apoptosis genes and Dcr2 ) have specific antiviral functions, and four groups including genes from the IMD, Toll, JAK/STAT and JNK pathway have both antibacterial and antiviral functions (Fig. 4d ). There are four groups of genes with unknown functions that encode proteins with immunoglobulin (Ig)-like, macroglobulin (Mg) domain, Sushi/SCR/CCP domain, and T/B cell-related features. We also found a large number of putative immune genes with predicate antibacterial function that were significantly upregulated in uninfected Ago2 −/− mutants as compared to WT mosquitoes at 4 days post blood feeding (Supplementary Fig. 6a and Supplementary Data 2 ), suggesting these groups of genes may not be induced by viral hyper-infection. At least eight caspase and apoptosis-related genes were upregulated, and one inhibitor of apoptosis gene ( IAP4 ) was downregulated in Ago2 −/− mutants at 4 dpi with MAYV (Supplementary Fig. 6b ). The upregulated genes included 6 caspase genes ( CASPS8 , CASPS9 , CASPS17 , CASPS18 , CASPS19 , and Dronc ), IMP-like IAP-antagonist Micheob_x-like protein ( IMP-like , AAEL014196) and nuclear apoptosis-inducing factor 1 ( NAIF1 , AAEL022840) genes. However, only one caspase gene ( CASPS8 ) was significantly upregulated in uninfected Ago2 −/− mutants as compared to WT mosquitoes (Supplementary Data 2 ). These data point to an upregulation of the apoptosis pathway in Ago2 − /− mutants in response to MAYV infection. Next, we measured overall caspase activity of Ago2 −/− and WT females using a caspase-3 assay kit, and our results showed that caspase activity was increased in the midguts and carcasses of Ago2 −/− mutants at 4 dpi with MAYV (Fig. 4e and Supplementary Fig. 6c ) and in DENV2-infected Ago2 −/− mutants at 14 dpi (Supplementary Fig. 6d ) when compared to WT mosquitoes. Transcript abundance analyses with qPCR confirmed that the expression of caspase and IMP-like genes was significantly induced in the midguts and carcasses of Ago2 −/− females at 4 dpi with MAYV (Fig. 4f and Supplementary Fig. 6e ) and in DENV2-infected Ago2 −/− females at 14 dpi (Supplementary Fig. 6f ). As compared to the WT mosquitoes, the midguts of the Ago2 −/− mutants had more apoptotic cells (by TUNEL staining) (Fig. 4g and Supplementary Fig. 6g ). The Ago2 −/− females exhibited a lower and higher probability of survival after MAYV infection (Fig. 4h ) when treated with an apoptosis inhibitor (Z-VAD-FMK) or inducer (PAC-1), respectively, and the virus titer was significantly increased or reduced in the inhibitor- or inducer-treated females (Fig. 4i ). These results together demonstrate that apoptosis is stimulated in Ago2 −/− mutants upon arbovirus infection, and these mutants may use an alternative antiviral mechanism against arboviral infection. Another group of upregulated immune genes have a predicted function related to the mammalian immune system, including B/T cell-mediated humoral/cellular immunity and complement. These genes were highly induced in Ago2 −/− mutants at 4 dpi with MAYV (Fig. 4j–k ). Overall, this stimulation of broad-spectrum antiviral genes in Ago2 −/− mutants upon arbovirus infection suggests that mosquitoes may engage other antiviral defense mechanisms to protect themselves from viral infection when the major antiviral siRNA pathway has been disrupted. Ago2 disruption impairs DNA repair and replication and reduces histone abundance GO and interacting network analyses of the downregulated genes showed that genes with functions related to DNA replication, repair, and metabolism were significantly downregulated in Ago2 −/− mutants at 4 dpi with MAYV (Fig. 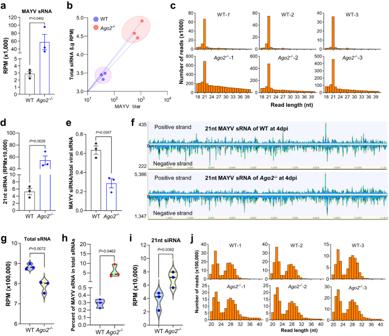Fig. 2: Impact ofAgo2disruption on production of MAYV- and mosquito-derived small RNAs. atotal number (reads per million mapped reads, RPM) of MAYV sRNAs inAgo2−/−mutants and WT mosquitoes at 4 days post-infection (dpi) as determined by sRNA sequencing. Three replicates were performed for each sample.bcorrelation between the abundance of sRNAs and titer of MAYV inAgo2−/−mutants and WT mosquitoes as determined by principal component analysis (PCA).cdistribution by length of sRNAs mapping to the MAYV genome.dnumber of 21-nt siRNAs mapped to the MAYV genome.ethe ratio of siRNA-sized (21 nt) MAYV reads to the total MAYV sRNA (18nt to 40nt) reads.fdistribution and the relative abundances of 21-nt MAYV siRNAs in the MAYV genome.gnumber of total sRNAs mapped to theAe. aegyptigenome.hpercent of MAYV sRNAs in the total sRNAs in mosquitoes.inumber of 21-nt siRNAs mapped to theAe. aegyptigenome.jlength distribution of the mosquito sRNAs.Pvalues were determined by using an unpaired two-sidedt-test (n= 3) with GraphPad Prism. Data are presented as mean ± SEM (a,dande). Source data are provided as a Source Data file. 5a and Supplementary Table 2 ), indicating that the DNA replication and repair mechanisms are significantly impaired in Ago2 −/− mutants. Then, we compared the expression of genes with predicated function in DNA damage response (DDR) that controls lesion detection and DNA repair [27] between Ago2 −/− mutants and WT mosquitoes. We found that most of the DDR genes that are involved in base excision repair (BER), double-strand break (DSB) repair, DNA mismatch repair (DMR) and nucleotide excision repair (NER) were downregulated in Ago2 −/− mutants in response to MAYV infection at 4 dpi (Fig. 5b, c and Supplementary Data 1 ), as compared to the WT mosquitoes. DMR and NER are the largest groups of the downregulated DNA repair genes. Most DDR genes were also downregulated and 8 of them were significantly downregulated in uninfected Ago2 −/− mutants as compared to WT mosquitoes at 4 days post blood feeding (Supplementary Fig. 7a and Supplementary Data 2 ), suggesting Ago2 disruption may have a direct impact on DNA repair. The downregulation of DDR genes was further confirmed by qPCR in Ago2 −/− females with or without MAYV infection at 4 dpi (Fig. 5d ), and with or without DENV2 infection at 14 dpi (Supplementary Fig. 7b ), as compared to the WT controls. Fig. 5: Transcriptomic analysis of DNA repair and histone genes in Ago2 −/− mutants upon MAYV infection and effect of histone reduction on virus infection and mosquito mortality. a interaction network illustrating downregulated gene families in Ago2 −/− mutants. The light color indicates small P -value (one-sided Fisher’s exact test), and the small size indicates few genes in the GO term. GOs related to DNA repair and replication are indicated by asterisks. b volcano plot illustrating fold changes in DNA repair genes ( DRG s) in Ago2 −/− mutants. c heatmap illustrating transcriptome changes in upregulated DRG s in Ago2 −/− mutants. d qPCR detecting expression of downregulated DRG s in Ago2 −/− carcasses. e fold enrichment of downregulated gene families in Ago2 −/− mutants. f downregulated histone genes in MAYV infected Ago2 −/− mutants. g volcano plot illustrating fold changes of histones-related genes in Ago2 −/− mutants. h overall histone level in MAYV infected Ago2 −/− and WT mosquitoes. i qPCR detecting expression of histone genes in carcasses of Ago2 −/− and WT mosquitoes at 4 days post-infection ( n = 4). j virus titer in histone dsRNA-injected WT females at 7 dpi as determined by plaque assay. Left: n = 35 (dsGFP), n = 28 (ds His2A ), n = 15 (ds His3 ) and n = 26 (ds His4 ). Righ: n = 29 (dsGFP) and n = 51 (ds His ). k virus titer in WT mosquitoes treated with histone deacetylase inhibitor Scriptaid (Scr), n = 20. l survival curves of MAYV-infected WT females that were fed with Scriptaid or DMSO in 10% sucrose solution. Data are represented as percents ± SE ( n = 3). qPCR detecting DRG expression ( m ) and histone expression ( n ) in WT females that were injected with ds His (mixture of dsRNAs of His2A , His3 and His4 ) or ds DRG (mixture of dsRNAs of cdk1 , RAD50, APE1 and KPNA2 ) at 3- and 7-days post injection, respectively. n = 4. P values were determined by a one-way ANOVA ( d , i ), an unpaired two-sided t -test ( h ), two-way ANOVA with multiple comparisons ( m and n ), a logrank (Mantel-Cox) test ( l ), or an unpaired two-sided Mann-Whitney test ( j , k ). Data are presented as mean ± SEM ( h , i , m and n ), and box and whiskers (Min to Max) ( d and j ) from 4 replicates. Source data are provided as a Source Data file. Full size image Taken together with our observation from the midgut TEM and TUNEL studies that the nuclei of the midgut cells in the mutant mosquitoes had an abnormal shape (Fig. 3d, e ) and underwent apoptosis and DNA fragmentation (Fig. 4g and Supplementary Fig. 6g ), our results here suggest that hyper-infection of arboviruses induces DNA damage in Ago2 −/− mutants, and Ago2 disruption impairs DNA repair mechanisms. Several histone genes were among those downregulated in Ago2 −/− mutants (Fig. 5e ), and the expression of at least 20 histone genes was significantly reduced by more than 2-fold in Ago2 −/− mutants at 4 dpi with MAYV (Fig. 5f ). Next, we compared the mRNA abundance of histones and histone-modifying enzyme genes between Ago2 −/− mutants and WT mosquitoes. Our results showed that the majority of these genes were downregulated in MAYV infected (Fig. 5g and Supplementary Data 1 ) and uninfected Ago2 −/− mutants (Supplementary Fig. 7c, d and Supplementary Data 2 ), and a reduction of up to 36.6% at 4 dpi with MAYV (Fig. 5h ) and 24.59% without infection (Supplementary Fig. 7e ), suggesting that impact of Ago2 disruption on histone abundance is independent of viral infection and downregulation of histones may be responsible for the impaired DNA replication and repair mechanisms in Ago2 −/− mutants. Next, we used qPCR to examine the expression of three histone core genes ( His2A , His3 and His4 ) that were significantly downregulated in the transcriptome of MAYV infected Ago2 −/− mutants. Our results showed that the mRNA abundance of these histone genes was significantly decreased in the midguts and carcasses of Ago2 −/− females, with or without MAYV infection (Fig. 5i and Supplementary Fig. 7f ), and with or without DENV2 infection (Supplementary Fig. 7g ), when compared to the corresponding WT mosquitoes, indicating that Ago2 disruption affects the expression of histones, independent of arbovirus infection. MAYV infection reduced the expression of histone genes in carcasses and midguts of the WT mosquitoes when compared to non-infected mosquitoes (Fig. 5i and Supplementary Fig. 7g ), suggesting that MAYV infection affects histone expression. To better understand the interaction between histones and arbovirus infection, we silenced three histone genes ( His2A , His3 , and His4 ) by injecting dsRNAs into the WT mosquitoes prior to virus infection. When compared to the GFP control, silencing of each histone gene significantly reduced the MAYV titer (Fig. 5j ). When the three histone genes were co-silenced, a significant 2.75-fold ( P < 0.0001) reduction in the MAYV titer was observed (Fig. 5j ). Furthermore, when the WT mosquitoes were treated with a histone deacetylase (HDAC) inhibitor (Scriptaid), which inhibits HDAC to remove acetyl groups from the lysine residues of histone and HDAC inhibitor treatment increases genome-wide histone acetylation [28] , they exhibited a significantly higher MAYV titer (Fig. 5k ) and lower survival rate (Fig. 5l ) than did those mosquitoes treated with a DMSO control. These data indicate that silencing of histones results in a decreased virus titer. To address whether histone downregulation leads to the impaired DDR in Ago2 −/− mutants, we co-silenced three histone genes ( His2A , His3 , and His4 ) in WT mosquitoes and then assayed mRNA abundance of DNA repair genes. Our results show that silencing of histone genes significantly affects mRNA abundance of all the DNA repair genes at 3 days post dsRNA injection and 7 of 8 DNA repair genes at 7 days post dsRNA injection (Fig. 5m ). On the other hand, co-silencing of DNA repair genes ( cdk1 , RAD50 , APE1 and KPNA2 ) reduces the mRNA abundance of His3 at 3 days post dsRNA injection but does not affect mRNA abundance of all three histone genes at 7 days post dsRNA injection even though silencing of DNA repair genes persists at that time point (Fig. 5n and Supplementary Fig. 8a ). Then, we silenced individual DNA repair gene and investigated its impact on histone gene mRNA abundance. We found that silencing of cdk1 had the most effect on histone gene mRNA abundance at 3 days post dsRNA injection (Supplementary Fig. 8b ). At 7 days post dsRNA injection, gene silencing was only persistent in RAD50 dsRNA-injected mosquitoes, but its silencing increased expression of His2A and His3 (Supplementary Fig. 8c ). Hence, the effect of DNA repair gene silencing on histone gene expression is inconclusive. Taken together, our data support the hypothesis that histone gene downregulation is the major reason for the observed defects in DNA replication and repair mechanisms in Ago2 −/− mutants. In summary, Ago2 disruption reduces the production of histones and compromises the DNA replication and repair mechanism in the arboviruses-infected mosquitoes. The downregulation of histone genes may play a protective role during arbovirus infection, likely through impairing the replication mechanism of the arboviruses. Ago2 disruption represses autophagy by altering histone abundance We found that Ref(2)P (polyubiquitin binding protein p62), which serves as a marker of autophagic flux in Drosophila [29] , [30] , was significantly upregulated, and two autophagy-related genes ( Atg ) were downregulated in the transcriptomes of Ago2 −/− mutants upon MAYV infection (Fig. 6a ). Most autophagy-related genes were also downregulated in uninfected Ago2 −/− mutants and one of them ( Atg10 ) was strongly downregulated (Supplementary Fig. 9a and Supplementary Data 2 ). Then, we used qPCR to examine the expression of a panel of Atg ( Atg5 , Atg7 , Atg10 , and Atg12 ), p62 and P53 , a transcription factor that transactivates a panel of Atg genes in Drosophila [31] , between Ago2 -/- mutants and WT mosquitoes in response to infection with different arboviruses. Our results confirmed the downregulation of Atg and P53 in Ago2 −/− mutants with or without MAYV infection at 4 dpi (Fig. 6b ), and with or without DENV2 infection at 14 dpi (Supplementary Fig. 9b ), as compared to the WT controls. We also observed downregulation of p62 in uninfected Ago2 −/− mutants as compared to the WT mosquitoes and MAYV infection increased p62 expression in Ago2 −/− mutants (Fig. 6b ). The protein levels of ATG8 and phosphatidylethanolamine (PE) of ATG8 (ATG8-PE), and P53 were also reduced in Ago2 −/− mutants as compared to the WT controls (Fig. 6c and Supplementary Fig. 9c–f ). These data suggest a less active autophagy pathway in Ago2 −/− mutants. Fig. 6: Effect of Ago2 disruption and histone loss on autophagy in mosquitoes upon MAYV infection. a upregulated p62 and downregulated autophagy-related genes ( Atg ) in the transcriptome of Ago2 −/− mutants. n = 3. b expression of p62 , P53 and Atg genes in the carcasses of Ago2 −/− and WT females at 4 days post-infection (dpi) with MAYV, as detected by qPCR. n = 4 biological replicates. c western blot showing protein levels of ATG8, ATG8-phosphatidylethanolamine (ATG8-PE) and P53 in Ago2 −/− and WT females at 4 dpi with MAYV; β-actin was used as a loading control. Western blots were repeated at least three times, and representative results are shown. Lysotracker Red (LTR) staining ( d ) showing the impairment of autophagy and LTR integrated density ( e ) in midguts of Ago2 −/− females at 4 dpi with MAYV. Nuclei were stained with DAPI (blue). n = 6 biologically independent samples. Autolysosomes (arrowheads) and autophagosomes (white arrows) were detected by TEM in the midguts of Ago2 −/− and WT females at 4 dpi ( f ) and 7 dpi ( g ) with MAYV. Yellow arrows indicate virions, and yellow arrowheads indicate cell debris. Abbreviations: Mi mitochondria, nc nucleus. n = 3 biologically independent samples. h virus titer in P53- or p62- dsRNA-injected WT females at 10 dpi with MAYV as determined by plaque assay. dsRNA for GFP was injected as a control. Data were presented as box and whiskers (Min to Max), n = 41 (dsGFP), n = 40 (ds P53 and ds p62 ). i survival curves of the MAYV-infected WT females that were fed with autophagy inhibitor 3-MA or inducer rapamycin (RAPA) or an equal amount of DMSO in 10% sucrose solution. Data were presented as percents ± SE ( n = 3). j qPCR detecting the expression of a panel of Atg genes in histone dsRNA-injected WT mosquitoes at 3 days post-injection and 4 days post-blood-feeding. n = 4 biological replicates. P values were determined by an unpaired two-sided t -test ( a , e and j ), one-way ANOVA for ( b ), an unpaired two-sided Mann-Whitney test for ( h ), and a logrank (Mantel-Cox) test ( i ). Data are represented as mean ± SEM ( a and b ). Source data are provided as a Source Data file. Full size image To further confirm the repressed autophagy in Ago2 −/− mutants, we used Lysotracker Red (LTR), a vital dye used for the detection of acidic organelles (including autolysosomes), to stain the midguts from Ago2 −/− and WT females at 4 dpi with MAYV. As compared to the WT mosquitoes, in which numerous LTR-positive dots accumulated in the midgut epithelium, the midguts of Ago2 −/− females showed a strongly reduced accumulation of LTR-positive cells (Fig. 6d ) and LTR integrated density (Fig. 6e ) upon MAYV infection. TEM was further used to document autophagy defects in the midgut cells of Ago2 −/− females. At 4 dpi with MAYV, many autophagosomes and autolysosomes were observed in the midgut cells of the WT mosquitoes, whereas the midgut cells of Ago2 −/− mutants exhibited a strong reduction in these autophagic structures, as well as numerous areas representing black cell debris/aggregates (Fig. 6f ). A large number of autophagosomes and autolysosomes were also present in the midgut cells of the WT mosquitoes at 7 dpi with MAYV (Fig. 6g ). Because of the strong cell lysis induced in Ago2 −/− mutants at 7 dpi with MAYV, we saw no autophagosomes or autolysosomes, but cell debris and black aggregates were present in both the cytoplasm and the nuclei (Fig. 6g ). Taken together, these results demonstrate that Ago2 disruption severely impairs the induction of autophagy upon arbovirus infection. To confirm the role of autophagy in inhibiting arbovirus infection in mosquitoes, we silenced P53 and p62 in the WT mosquitoes prior to infection and determined the virus titer in the silenced mosquitoes. The results showed that the MAYV titer was significantly elevated in the P53 -silenced mosquitoes and suppressed in the p62 -silenced mosquitoes (Fig. 6h ). When Ago2 −/− mutants were treated with the autophagy inhibitor 3-MA or an inducer, rapamycin, they exhibited a significantly lower or higher probability of survival, respectively, upon MAYV infection (Fig. 6i ). These data indicate that autophagy plays a role in preventing mosquito death during arbovirus infection by inhibiting viral infection. The regulation of autophagy is linked to histone modification and altered histone abundance in mammals [32] , [33] . To test the effect of histone loss on autophagy in mosquitoes, we silenced three histone genes ( His2A , His3 , and His4 ) by injecting a mixture of dsRNAs for these genes into the WT mosquitoes and monitoring the Atg expression by qPCR in the silenced mosquitoes. As compared to the GFP control, silencing the histone genes significantly reduced the expression of a panel of autophagy genes ( Atg5 , Atg7 , Atg10 , and Atg12 ) in both sugar-fed and blood-fed mosquitoes (Fig. 6j ), and these results were correlated with the silencing efficiency of the histone genes (Supplementary Fig. 9g ). As compared to the sugar-fed mosquitoes, the blood-fed mosquitoes exhibited a significantly higher expression of Atg5 and Atg10 in the GFP control mosquitoes, but not in the histone -silenced mosquitoes. In summary, Ago2 disruption significantly repressed the autophagy pathway in mosquitoes, most likely by affecting histone production, and this reduced autophagy promoted mosquito death by hampering the removal of damaged cell aggregates in the arbovirus-hyper-infected mosquitoes. A proposed model of arbovirus-induced mosquito death mechanism We propose a working model to summarize our findings and to explain an arbovirus-induced mosquito death mechanism in Ago2 −/− mutants (Fig. 7 ): (1) Ago2 disruption does not affect the biogenesis of small RNA but impairs the arboviral RNA degradation through a defective siRNA pathway in Ae. aegypti ; (2) Ago2 disruption leads to arbovirus hyper-infection of mosquitoes, which is accompanied by cell lysis and results in mortality; (3) Ago2 disruption influences the production of histones, which represses the autophagy and DNA repair mechanism in arboviruses-hyper-infected mosquitoes. (4) hyper-infection by arboviruses and defect in DNA repair along with cytoplasmic degradation promote mosquito death. Fig. 7 A proposed model summarizing arboviruses-induced death in Ago2 -deficient Ae. aegytpi . Full size image Here we show that the Ae. aegypti Ago2 is essential for controlling arbovirus infection, and thereby an important regulator of mosquito disease transmission. We describe a mechanism to account for the lethality caused by arbovirus infection in siRNA pathway-defective mosquitoes ( Ago2 −/− mutants), in which hyper-infection leads to lysis of mosquito cells and damage to tissues, while at the same time the DNA repair/replication mechanism and elimination of damaged and dysfunctional cytoplasmic materials are severely impaired. Further analysis revealed that the reduced abundance of histones in Ago2 −/− mutants may compromise their DNA repair mechanism and autophagy. Arbovirus-induced mortality was also observed in Dicer2 −/− mutant mosquitoes that also have an impaired siRNA pathway, but mortality of Dicer2 −/− mutants differs between infections with different arboviruses; e.g. mortality upon chikungunya virus (CHIKV) infection vs no significant mortality upon DENV3 infection [34] and high mortality upon Sindbis virus (SINV) infection vs low mortality upon yellow fever virus (YFV) infection [35] . It appears that infections by alphaviruses (CHIKV, SINV and MAYV) induces a higher mortality in siRNA-deficient mosquitoes as compared to flaviviruses (DENV2, DENV3, ZIKV and YLV). It is impossible to quantitatively compare arbovirus-induced mortality in Ago2 −/− and Dicer2 −/− mutants because of differences in arboviruses, viral titers, infection methods (systemic injection vs blood feeding) used in these independent studies. In the baculovirus-insect system, infection alters insect physiology and behavior [36] and usually causes lethality in the larval stages of some lepidopterans, mosquitoes, and sawflies [37] . For example, in the fall armyworm ( Spodoptera frugiperda ), larval infection with baculovirus blocks molting as a result of the production of a viral enzyme, ecdysteroid UDP-glucosyltransferase (EGT), which prevents larval molting by inactivating ecdysone [38] . In contrast to the baculoviruses-insect system, infection with arboviruses in mosquitoes is nonpathogenic, preventing vaccinated strains of arboviruses from potentially being used as biological insecticides for mosquito control, as baculoviruses are. Our results here show that impairment of the siRNA pathway renders mosquitoes hypersensitive to infection by arboviruses and converts a nonpathogenic infection with arboviruses in mosquitoes into a lethal infection. Importantly, the vector competence (transmission potential) of arboviruses in Ago2 −/− mutants was significantly lower than that of WT mosquitoes despite the fact that the mutant mosquitoes had a higher titer of arboviruses, which suggests that this type of siRNA pathway disruption could be explored for the development of novel arbovirus transmission-blocking strategies. Our results demonstrate that the siRNA pathway is an essential determinant of persistent infection by arboviruses in mosquitoes. Unlike vertebrates with a well-developed immune system, insects lack adaptive or acquired immune responses but have constitutive and induced systemic and local innate immune defenses against pathogen infection [39] , [40] . In Drosophila , the siRNA pathway is considered a constitutive defense system against virus infection, whereas the other innate immune pathways are inducible by infection with various pathogens [20] . Here we also show that when the siRNA pathway is impaired, other conserved immune signaling cascades, including the Toll and apoptosis pathways, are induced upon virus infection or other stresses and injuries and may play a role in defending against viral infection. A siRNA pathway deficiency appears to be compensated by complementary antiviral response comprising diverse defense systems that, however, will be inadequate to suppress virus infection to a tolerable level. In addition to induction of classical innate immune signaling, hyper-infection of arboviruses also stimulates induction of immune genes with macroglobulin and Sushi/SCR/CCP domains, and these genes have predicted functions related to mammalian immune signaling, including B/T cell-mediated humoral/cellular immunity and complement, but their antiviral role has not been explored in mosquitoes or other insects. We report that Ago2 disruption severely impairs the degradation of viral dsRNA, resulting in high infection intensities in Ago2 −/− mutants, which demonstrates the essential role of Ago2 in the mosquito siRNA pathway. Meanwhile, the production of viral small interfering RNAs (vsiRNAs) is increased in Ago2 −/− mutants, indicating that Ago2 disruption does not affect the endonuclease activity of Dcr2 to process viral dsRNA into 21-nt vsiRNA as shown in Drosophila [41] , [42] . Despite the high amount of vsiRNA in Ago2 −/− mutants, their failure to form RNA-induced silencing complexes (RISCs) because of a lack of Ago2 prevents the RISC-mediated degradation of the viral dsRNA. In our previous study, we have shown that overexpression of Dcr2 in mosquito midguts significantly reduces the production of vsiRNA as a result of the low viral titer in transgenic mosquitoes [43] , indicating that the production of vsiRNA is dependent on both the arbovirus titer and Dcr2 activity. Therefore, Dcr2 activity appears to be independent of Ago2, and Dcr2 functions upstream of the siRNA production. According to our findings, the abundance of mosquito 21nt-siRNAs is also increased in Ago2 −/− mutants as compared to WT mosquitoes, suggesting that Ago2 disruption may adversely affect the degradation of endogenous mosquito dsRNAs. Taken together, our results show that Ago2 functions downstream of the siRNA pathway in mosquitoes and plays key roles in degrading endogenous (mosquito) and exogenous (arbovirus) dsRNAs. DNA repair and replication mechanisms and histone abundance are significantly affected by arbovirus infection in Ago2 −/− mutants. Considering the role of histones in mediating DNA repair and replication [44] , [45] , [46] , the impaired DNA repair and replication in Ago2 −/− mutants may be a result of the decreased abundance of histones. Histone loss in Ago2 −/− mutants might be caused by hyper-infection of arboviruses and the resulting induction of DNA damage, as has been reported in in yeast [47] . However, a reduced expression of histone genes when compared to WT mosquitoes was also observed in Ago2 −/− mutants in the absence of arbovirus infection. These data indicate that Ago2 disruption may have a direct impact on histone production in mosquitoes, suggesting that Ago2 may play a role in modifying nucleolus organization through affecting histone production and modification, as has been reported in Drosophila and mammals, in which Ago2 is involved in chromatin topology [19] and modification [48] , [49] , and chromatin changes can be modulated by histone variants and modification [50] , [51] , [52] . Autophagy is a highly conserved process in eukaryotic cells for maintaining cellular and tissue homeostasis by degrading damaged organelles and unfolded proteins, and this pathway plays a pivotal role in cells by allowing them to recycle or clear cytoplasmic organelles or cytosolic aggregates under conditions of starvation or other types of cellular stress [53] , [54] . Autophagy can also be stimulated by infection with intracellular pathogens, including viruses, and it plays a protective role in cells during pathogen infection in Drosophila [55] , [56] , [57] . In mosquito cells, infection with DENV2 and CHIKV induces autophagy [58] , and treatment with the autophagy inducer rapamycin can activate the autophagy pathway to defend the mosquitoes against DENV infection [59] . Our results now show that Ago2 disruption in adult mosquitoes significantly represses autophagy and enhances mosquito death most likely because the cells fail to clear the damaged organelles and other cytoplasmic components that are produced by hyper-infection with arboviruses. The repressed autophagy may result from the impaired histone production in Ago2 −/− mutants, which is consistent with the role of histones in controlling autophagic flux in mammals, where reduced histone modification and histone variants are associated with dysfunction in autophagic processes and sustained autophagy [32] , [33] , [60] . Taken together, our data strongly support the conclusion that autophagy plays a protective role during arbovirus infection in Ae. aegypti by degrading damaged cell aggregates and inhibiting viral infection, and Ago2 disruption weakens this protective role by affecting histone production and rendering the mosquitoes vulnerable to viral infection. Ethics statement This study was carried out in accordance with the recommendations in the Guide for the Care and Use of Laboratory Animals of the National Institutes of Health, the Animal Care and Use Committee (ACUC) of the Johns Hopkins University, and the institutional Ethics Committee (permit number: M006H300). The IACUC committee approved the protocol. Mice were only used for mosquito rearing. Commercial, anonymous human blood was used for virus infection assays in mosquitoes, and informed consent was therefore not applicable. Mosquitoes The germline Cas9 -expressed Ae. aegypti line ( Cas9 ) [61] was shared by Dr. Omar Akbari. All the mosquitoes used in these experiments, including wildtype (Liverpool strain), Cas9 , and Ago2 knockout mutant lines were reared at 27 °C under 85% relative humidity with a 12 h light/12 h dark cycle in a walk-in chamber in the Johns Hopkins Malaria Research Institute. Mice (6 to 12 weeks old) were used for blood feeding and colony maintenance and reared at 27 °C under 50% relative humidity with a 12 h light/12 h dark cycle. Generation of Ago2 knockout mutant lines using CRISPR/Cas9 Guide RNA (gRNA) design and synthesis have been described [62] . In brief, the Ago2 gRNAs were designed using the chopchop CRISPR/Cas9 ( https://chopchop.cbu.uib.no/ ). Each of two gRNAs separated by around 300-bp were designed to target the same Ago2 exon sequence to achieve a large mutation. The double-stranded DNA templates for each gRNA were generated by template-free PCR, and the purified PCR products were in vitro-transcribed using a HiScribe™ T7 Quick High Yield RNA Synthesis Kit (NEB). Following transcription, the gRNAs were purified using a RNeasy kit (Qiagen), eluted with nuclease-free water, and stored at −80 °C. For embryo injection, each gRNA was diluted to 100 ng/μl with E-Toxate™ Water (Sigma) and injected into Cas9 embryos according to our previously established protocol [62] . 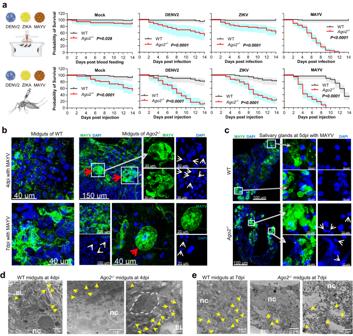Fig. 3: Effect of arbovirus infection on mosquito death and tissue/cell damage inAgo2−/−mutants. asurvival curves ofAgo2−/−and wild-type (WT) females that ingested a blood meal containing DENV2, ZIKV, or MAYV or were mock-infected (given C6/36 cell culture medium), or were injected with DENV2, ZIKV, or MAYV or mock-infected medium.Pvalues betweenAgo2−/−mutants and WT mosquitoes were determined using the logrank (Mantel-Cox) test. Each experiment comprised at least three biological replicates. The error bands were indicated by the shaded region. IFA detection with the anti-MAYV monoclonal antibody (green) of MAYV in midguts (b) and salivary glands (c) ofAgo2−/−and WT females at various days post-infection (dpi). Nuclei were stained with DAPI (blue). The zoomed areas are indicated as white boxes and arrows. White arrows indicate abnormal nuclei, and red arrows indicate strong fluorescence with a “ball” shape. Ultrastructural TEM images showing cross-sections of midgut tissue ofAgo2−/−mutants and WT mosquitoes at 4 dpi (d) and 7 dpi (e) with MAYV. Yellow arrows indicate individual virion; white dotted lines outline a cluster of virions. Scale bars are indicated on each image. Abbreviations: BL basal lamina, nc nucleus. The IFA and TEM images in (b–e) are representative of three biologically independent samples. Source data are provided as a Source Data file. A leg PCR was used to identify mutations in the surviving G0 adults using a pair of primers ~100 bp outside of each gRNA (Supplementary Table 3 ). The mutation was identified by an extra band on a 2% agarose gel when compared to the Cas9 line. The mutated G0 was crossed back to Cas9 line, and mutation of their offspring (G1) was identified by leg PCR. Each mutated G1 male or female was individually outcrossed with the corresponding Cas9 female or male to establish various mutant lines. After another four generations, the heterozygotes were in-crossed. The homozygous mutant lines were identified by leg PCR and confirmed by DNA Sanger sequencing. The homozygous mutant females were also crossed to the WT males for another six generations to establish the WT-genetic background of the Ago2 mutant lines. Virus infection, transmission, and titration Virus infection of mosquitoes and plaque assays were performed as previously described [63] : MAYV (Iquitos, IQT), ZIKV (Cambodia, FSS13025) or DENV serotype 2 (New Guinea C strain, DENV2) was propagated in C6/36 cells. 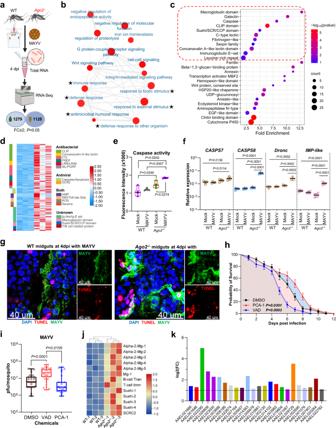Fig. 4: Transcriptomic analysis of antiviral immune signaling inAgo2−/−mutants upon MAYV infection. aflowchart illustrating the design and outcome of RNAseq experiments comparing transcriptome changes inAgo2−/−mutants and WT mosquitoes. DE genes, differentially expressed genes.n= 3 biological replicates.binteraction network illustrating the upregulated gene families inAgo2−/−mutants. The light color indicates the smallP-value (one-sided Fisher’s exact test), and the small size of the bubble indicates the few genes in the GO term. The immunity- and defense-related GOs are indicated by asterisks.cfold enrichment of the significantly upregulated gene families inAgo2−/−mutants. The immunity-related gene families are outlined red.dheatmap illustrating transcriptome changes in the upregulated immunity genes inAgo2−/−mutants.edetection of caspase activity in midguts ofAgo2−/−and WT females. Data are presented as mean ± SD (n= 4).fconfirmation by qPCR of the upregulated expression of caspase and apoptosis genes in midguts ofAgo2−/−females. Data are presented as mean ± SD (n= 4).gTUNEL assay to detect apoptotic cells (red) in midguts ofAgo2−/−and WT females. MAYV antigen is indicated by green, and nuclei are in blue.hsurvival curves for the MAYV-infected WT females that were fed with apoptosis inducer PAC-1 or apoptosis inhibitor Z-VAD-FMK (VAD) or an equal amount of DMSO in 10% sucrose solution. Data are presented as percents ± SE (n= 3).ivirus titer in WT females treated with PAC-1 or VAD at 7 dpi with MAYV. Data were presented as box and whiskers (Min to Max),n= 30.jupregulated immune genes related to B-cell, T-cell, complement (Suchi), or macroglobulin (Mg) inAgo2−/−mutants.kupregulated immunoglobulin (Ig)-like genes inAgo2−/−mutants.Pvalues were determined by one-way ANOVA (eandf), an unpaired two-sided Mann-Whitney test (i), or a logrank (Mantel-Cox) test (h). Source data are provided as a Source Data file. The virus-infected cell culture medium was harvested and mixed with an equal volume of commercial human blood supplemented with 10% human serum containing 10 mM ATP. One-week-old females were starved overnight and transferred into a small cup, then fed for 30 min with the blood-virus mixture at 37 °C on a single glass artificial feeder. Fully engorged females were selected and maintained on 10% sterile sucrose solution. Each experiment had at least two biological replicates, and each replicate included at least 20 individual females. Viral transmission in mosquitoes was assayed using an artificial glass feeder according to our previously established method [62] . In brief, a cup of eight mosquitoes were fed on a sterilized glass feeder with 200 μl of feeding solution (equal volumes of human serum and DMEM together with 10 mM ATP [final concentration]) for 30 min at 5 dpi with MAYV. Forced salivation was used to collect saliva from individual females [62] , and more than 20 mosquitoes were assayed for each strain. The virus titers in the feeding solution and individual saliva were determined by plaque assay. At least two biological replicates were performed for each experiment, and the data were pooled from different replicates and used for generating graphs. Plaque assays were used to determine the virus titer as previously described [21] , [63] . In brief, mosquitoes were homogenized in 300 μl of DMEM with a Bullet Blender (Next Advance Inc., Averill Park, NY, USA) with glass beads. They were then centrifuged at 10,000 g for 3 min, and 20 μl of the filtered supernatants were used for plaque assays in 24-well plates, using BHK 21 cells for DENV2 and ZIKV and Vero cells for MAYV. The plates were incubated for 2 days (MAYV), 4 days (ZIKV), or 5 days (DENV2), and then the plaques were visualized by staining with 1% crystal violet and counted under a microscope. At least two biological replicates were performed, and the data were pooled from different replicates and used for generating graphs. Differences in virus titer and prevalence of infection between different samples were compared by using a non-parametric two-sided Mann-Whitney U-test and Fisher’s exact test, respectively. Gene silencing assays and qRT-PCR dsRNA was synthesized using a HiScribe T7 in vitro transcription kit (New England Biolabs) with gene-specific primers (Supplementary Table 3 ) and purified using a RNeasy kit (Qiagen). Four- or five-day-old females were cold-anesthetized and injected intrathoracically by using the Nanoject II injection system (Drummond Scientific) with about 0.5 μg of dsRNA per mosquito. Two days after dsRNA injection, the females were given a blood-virus mixed meal for infection. dsGFP-injected mosquitoes were used as a control. The gene silencing efficiency was monitored by qPCR. At least three replicates were performed. The embryos of WT and Ago2 knockout mutants were injected with 1 μg/μl of dsRNA, and larvae hatched from dsRNA-injected eggs were photographed. dsGFP-injected eggs were used as a control. At least 100 eggs were injected from each condition, and two biological replicates were performed. Total RNA was extracted from mosquitoes or tissues with Trizol reagent (Invitrogen, Carlsbad, CA, USA). First-strand cDNA was synthesized using a QuantiTect Reverse Transcription Kit (Qiagen, Hilden, Germany). qPCR amplification was performed with gene-specific primers (Supplementary Table 3 ) on a StepOnePlus Real-Time PCR System (Applied Biosystems, Warrington, UK). The relative abundance of the gene transcripts was normalized and calculated by comparison to the ribosomal protein S7 gene as an endogenous reference using the 2 −ΔCT or 2 −ΔΔCT method. Each sample had at least three independent biological replicates. The significance ( P -values) between samples was determined by using an unpaired two-sided t -test with GraphPad Prism. Western blotting, immunofluorescence (IFA), and TUNEL assays Total proteins were extracted from mosquitoes with RIPA extraction buffer (Thermo Scientific) supplemented with a 1% cOmplete™ Protease Inhibitor Cocktail (Roche Applied Science). A total of 20 µg of total protein were used in blotting as described previously [62] . Primary antibodies for western blotting were as follows: Ae. aegypti anti-ATG8 polyclonal antibody [64] (a gift from Dr. Alexandra Raikhel) and anti-P53 rabbit polyclonal antibody (ABclonal, cat#: A3185). HRP-conjugated anti-rabbit (Cell Signaling Technology) secondary antibody was used and then detected using Amersham ECL Prime Western Blotting detection reagents. Anti-β-actin-peroxidase antibody (Sigma, cat#: A5316) was used to detect the loading control. All western blotting experiments were repeated at least three times, and representative results are shown in the figures. IFA for midgut and salivary gland samples followed the previously described protocol [62] . Anti-MAYV E2 antibody (Sigma, cat#: MABF3046) or mouse hyperimmune ascitic fluid specific for DENV2 [65] was used to detect MAYV or DENV2 antigen, respectively, and the secondary antibody was AlexaFluor 488 goat anti-mouse IgG (Invitrogen). For TUNEL staining, the TMR red reaction mixture (Roche Applied Science) was incubated with the secondary antibody. 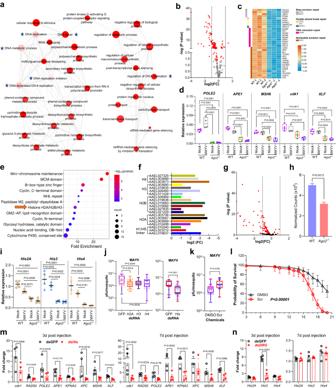Fig. 5: Transcriptomic analysis of DNA repair and histone genes inAgo2−/−mutants upon MAYV infection and effect of histone reduction on virus infection and mosquito mortality. ainteraction network illustrating downregulated gene families inAgo2−/−mutants. The light color indicates smallP-value (one-sided Fisher’s exact test), and the small size indicates few genes in the GO term. GOs related to DNA repair and replication are indicated by asterisks.bvolcano plot illustrating fold changes in DNA repair genes (DRGs) inAgo2−/−mutants.cheatmap illustrating transcriptome changes in upregulatedDRGs inAgo2−/−mutants.dqPCR detecting expression of downregulatedDRGs inAgo2−/−carcasses.efold enrichment of downregulated gene families inAgo2−/−mutants.fdownregulated histone genes in MAYV infectedAgo2−/−mutants.gvolcano plot illustrating fold changes of histones-related genes inAgo2−/−mutants.hoverall histone level in MAYV infectedAgo2−/−and WT mosquitoes.iqPCR detecting expression of histone genes in carcasses ofAgo2−/−and WT mosquitoes at 4 days post-infection (n= 4).jvirus titer in histone dsRNA-injected WT females at 7 dpi as determined by plaque assay. Left:n= 35 (dsGFP),n= 28 (dsHis2A),n= 15 (dsHis3) andn= 26 (dsHis4). Righ:n= 29 (dsGFP) andn= 51 (dsHis).kvirus titer in WT mosquitoes treated with histone deacetylase inhibitor Scriptaid (Scr),n= 20.lsurvival curves of MAYV-infected WT females that were fed with Scriptaid or DMSO in 10% sucrose solution. Data are represented as percents ± SE (n= 3). qPCR detectingDRGexpression (m) and histone expression (n) in WT females that were injected with dsHis(mixture of dsRNAs ofHis2A,His3andHis4) or dsDRG(mixture of dsRNAs ofcdk1,RAD50, APE1andKPNA2) at 3- and 7-days post injection, respectively.n= 4.Pvalues were determined by a one-way ANOVA (d,i), an unpaired two-sidedt-test (h), two-way ANOVA with multiple comparisons (mandn), a logrank (Mantel-Cox) test (l), or an unpaired two-sided Mann-Whitney test (j,k). Data are presented as mean ± SEM (h,i,mandn), and box and whiskers (Min to Max) (dandj) from 4 replicates. Source data are provided as a Source Data file. DAPI was used to stain the nuclei. Samples were viewed and photographed under a Zeiss LSM700 confocal microscope at the Johns Hopkins University School of Medicine Microscope Facility. Caspase activity Midguts and carcasses were dissected from mosquitoes and homogenized in cold cell lysis buffer from the EnzChek caspase-3 assay kit. After centrifugation at 10,000 g for 10 min at 4 °C, the supernatants were transferred to a new tube. 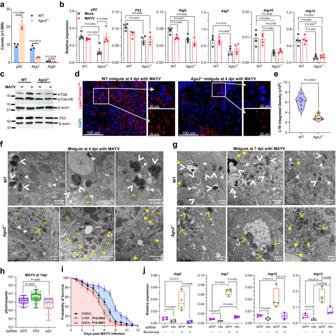Fig. 6: Effect ofAgo2disruption and histone loss on autophagy in mosquitoes upon MAYV infection. aupregulatedp62and downregulated autophagy-related genes (Atg) in the transcriptome ofAgo2−/−mutants.n= 3.bexpression ofp62,P53andAtggenes in the carcasses ofAgo2−/−and WT females at 4 days post-infection (dpi) with MAYV, as detected by qPCR.n= 4 biological replicates.cwestern blot showing protein levels of ATG8, ATG8-phosphatidylethanolamine (ATG8-PE) and P53 inAgo2−/−and WT females at 4 dpi with MAYV; β-actin was used as a loading control. Western blots were repeated at least three times, and representative results are shown. Lysotracker Red (LTR) staining (d) showing the impairment of autophagy and LTR integrated density (e) in midguts ofAgo2−/−females at 4 dpi with MAYV. Nuclei were stained with DAPI (blue).n= 6 biologically independent samples. Autolysosomes (arrowheads) and autophagosomes (white arrows) were detected by TEM in the midguts ofAgo2−/−and WT females at 4 dpi (f) and 7 dpi (g) with MAYV. Yellow arrows indicate virions, and yellow arrowheads indicate cell debris. Abbreviations: Mi mitochondria, nc nucleus.n= 3 biologically independent samples.hvirus titer inP53-orp62-dsRNA-injected WT females at 10 dpi with MAYV as determined by plaque assay. dsRNA for GFP was injected as a control. Data were presented as box and whiskers (Min to Max),n= 41 (dsGFP),n= 40 (dsP53and dsp62).isurvival curves of the MAYV-infected WT females that were fed with autophagy inhibitor 3-MA or inducer rapamycin (RAPA) or an equal amount of DMSO in 10% sucrose solution. Data were presented as percents ± SE (n= 3).jqPCR detecting the expression of a panel ofAtggenes in histone dsRNA-injected WT mosquitoes at 3 days post-injection and 4 days post-blood-feeding.n= 4 biological replicates.Pvalues were determined by an unpaired two-sidedt-test (a,eandj), one-way ANOVA for (b), an unpaired two-sided Mann-Whitney test for (h), and a logrank (Mantel-Cox) test (i). Data are represented as mean ± SEM (aandb). Source data are provided as a Source Data file. 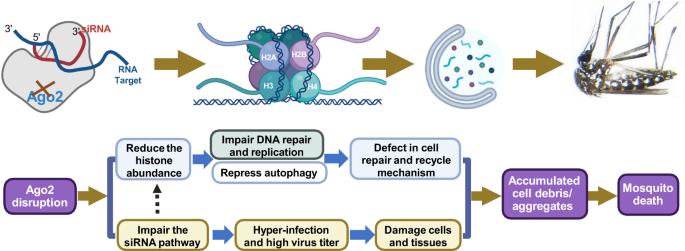Fig. 7 A proposed model summarizing arboviruses-induced death inAgo2-deficientAe. aegytpi. Caspase activity assays were performed using the synthetic fluorescent substrate Z-DEVD-AMC, and the reactions were carried out according to the protocol of the EnzChek caspase-3 assay kit. The fluorescence (excitation/emission, ~342/441 nm) was measured every 5 min for 30 min using a plate reader. At least four technical repeats were performed, with three biological replicates. Data from one biological replicate were used for generating the graph. LTR assay Midguts were dissected from Ago2 mutant and WT mosquitoes in cold PBS and then stained with 0.1 μM LysoTracker Red DND-99 (Invitrogen) for 5 min. Samples were immediately viewed using under a fluorescence microscope with an excitation/emission of 577/590 nm. Samples were also fixed in 4% paraformaldehyde for 30 min at room temperature. After three washes with PBS, midgut samples were placed individually on a glass slide and mounted with Fluoromount-G with DAPI (Electron Microscopy Sciences Hatfield, PA, USA). Images were obtained using a Zeiss LSM700 confocal microscope. Transmission electron microscopy (TEM) Midguts were dissected and fixed overnight at 4 °C in 2% glutaraldehyde and 2% paraformaldehyde in 0.1 m cacodylate buffer (Sigma Aldrich, St. Louis, MO). Secondary fixation was performed using 1% osmium tetroxide (Ted Pella, Inc. Redding, CA) in 100 mM sodium cacodylate. After dehydration in an ethanol-acetone series, midguts were infiltrated with Epon resin. Midgut sections were cut to a thickness of 85 nm with a diamond knife on the Reichert-Jung Ultracut E ultramicrotome and stained with 2% uranyl acetate in 50% methanol and 0.4% lead citrate. Images were captured at 120 kV on a 16-megapixel CMOS camera on a Talos L120C G2 Transmission Electron Microscope (Thermo-Fisher) at the Johns Hopkins University School of Medicine Microscopy Core. RNA-Seq and small RNA library preparation, sequencing, and bioinformatics analysis Total RNA was extracted from 10 females of MAYV-infected or uninfected WT (Liverpool strain) and Ago2 −/− mutants at 4 dpi, or DENV2-infected cas9 (parental line) and AgoN −/− mutants at 2 and 7 dpi per sample using TRIzol reagent (Invitrogen, Carlsbad, CA), and three independent biological replicates were included for each sample. An Illumina sequencing library was constructed from total RNA using poly(A) enrichment of the mRNA for each RNA sample according to the manufacturer’s instructions and sequenced by Novogene Co., LTD (Beijing, China) on the Illumina platform with paired-end 150 bp (PE 150). Data were deposited into NCBI’s Sequence Read Archive (SRA) (PRJNA889408). Raw data in FASTQ format were processed to remove reads containing adapters, reads containing ploy-N, and low-quality reads, and clean reads were aligned to the Ae. aegypti genome (VectorBase-57). FeatureCounts was used to quantify transcript abundance in each sample using the gene annotation obtained from VectorBase. Differentially expressed (DE) genes between Ago2 −/− mutants and the WT mosquitoes were identified with DESeq2. Gene ontology (GO) and -fold enrichment of the DE genes were analyzed using the built-in program in Vectorbase or ShinyGO ( http://bioinformatics.sdstate.edu/go/ ). The interaction networks of the DE genes were generated with Revigo ( http://revigo.irb.hr/ ) [66] and modified by Cytoscape [67] . The small RNA libraries were prepared from the total RNA using a Perkin Elmer Small NextFlex v3 according to the standard protocol. The small RNA sequencing was performed on an Illumina NovaSeq6000 with a paired-end 100 bp at the Institute for Genome Sciences, University of Maryland School of Medicine. The paired reads were aligned to the DENV2 or MAYV genome or mosquito virus genome [68] using Geneious Prime or to the Ae. aegypti genome (VectorBase-57) using HISAT2 at Usegalaxy ( https://usegalaxy.org/ ). Pharmacological treatment, virus injection, and mortality assays Newly emerged adult females were placed in a cup and were fed with 10% sterile sucrose solution containing 20 mM of apoptosis inducer PAC-1 (Selleck), apoptosis inhibitor Z-VAD-FMK (Selleck), autophagy inducer rapamycin (Millipore), autophagy inhibitor 3-MA (Selleck), or histone deacetylase (HDAC) inhibitor Scriptaid (Millipore). An equivalent amount of DMSO was used as a control. All chemicals were changed daily. On the fifth day of pharmacological treatment, mosquitoes were infected with the various viruses through blood feeding. The viruses were injected intrathoracically into the mosquitoes by using the Nanoject II injection system (Drummond Scientific) with 69 nl of MAYV (1.8 × 10 8 pfu/ml), DENV2 (10 7 pfu/ml) or ZIKV (10 7 pfu/ml) per mosquito. An equivalent volume of C6/36 cell culture medium was injected as a control. Each experiment had at least two biological replicates, and each replicate included at least 20 individual females. The number of dead mosquitoes in each cup was recorded daily. Statistical significance was determined by Kaplan-Meier survival analysis with pooled data from different replicates by using GraphPad Prism software, and the P -values were determined by the logrank (Mantel-Cox) test. Reporting summary Further information on research design is available in the Nature Portfolio Reporting Summary linked to this article.